Atomically resolved tomography to directly inform simulations for structure–property relationships Microscopy encompasses a wide variety of forms and scales. So too does the array of simulation techniques developed that correlate to and build upon microstructural information. Nevertheless, a true nexus between microscopy and atomistic simulations is lacking. Atom probe has emerged as a potential means of achieving this goal. Atom probe generates three-dimensional atomistic images in a format almost identical to many atomistic simulations. However, this data is imperfect, preventing input into computational algorithms to predict material properties. Here we describe a methodology to overcome these limitations, based on a hybrid data format, blending atom probe and predictive Monte Carlo simulations. We create atomically complete and lattice-bound models of material specimens. This hybrid data can then be used as direct input into density functional theory simulations to calculate local energetics and elastic properties. This research demonstrates the role that atom probe combined with theoretical approaches can play in modern materials engineering. Atomic-scale microscopy enables the characterization of incredibly small and complex structures, and increasingly is the gateway for advances in materials technology. However, it is the complementary development of computational materials science that has been key to unlocking our understanding of the mechanisms by which atomic architectures directly impact the properties and behaviour of materials. Impressive inroads have been made in materials characterization over the last decade, particularly through continued advances in the capabilities of electron microscopy, most notably the efforts in high-resolution aberration-corrected transmission electron microscopy (TEM) [1] and scanning TEM [2] and the development of tomographic TEM techniques [3] . Atom probe tomography (APT) is a very different three-dimensional (3D) microscopy concept, but one that is rapidly rising in prominence [4] , [5] , [6] . On the basis of sequential field evaporation of individual ions from the surface of a sharp needle-shaped specimen, APT provides a highly accurate elementally resolved, atom-by-atom 3D image of a specimen encompassing hundreds of millions of atoms ( Supplementary Fig. 1 ). The data generated by APT is of a format almost identical to that exploited by many types of computer simulations. Indeed, one of the necessary precursors to carrying out atomistic modelling is to have the initial microstructure configurations as close as possible to real structures [7] . In constitutive modelling of inhomogeneous systems, grid points or supercells are often employed to represent different parts of the microstructures. A fundamental problem with such an approach is that the actual microstructures may differ significantly from simulated ones because of the presence of non-uniform distributions of crystal orientation, and morphology [8] . APT has previously been used to bridge this gap between experimental microscopy and atomistic simulation. Many studies have demonstrated this potential by using atom probe data to indirectly inform various flavours of computational materials science, including Monte Carlo (MC) simulations [9] , [10] , [11] , [12] , molecular dynamics (MD) [13] and density functional theory (DFT) [14] , [15] , [16] , [17] , [18] , [19] . In each case, APT offers valuable information to construct relevant models, and the simulated results can subsequently be compared with experiments. However, although APT reconstructions represent a highly spatially resolved atomistic representation of a material system, this data remains both imperfect and significantly incomplete. This is key since it prevents APT data from being seeded directly into theoretical models and simulations, and thus prevents the full potential of its information from being realised. The 3D spatial resolution of APT can be extremely high [20] , [21] , however, the location of atoms in the reconstructed image is not exact. As a result, in the analysis of crystalline materials, atoms are offset from their true positions on the lattice. Further, due to the incorporation of multi-channel plates in the design of the position-sensitive detectors, a significant proportion of ions striking the detector are simply omitted from the final reconstructed image. This process is often considered stochastic and independent of the identity of the incident ion. The term detection efficiency refers to the fraction of ions that are successfully detected, and in most commercial instruments has an estimated value of ε ≈0.37–0.57. Imperfect spatial resolution and detection efficiency are two of the most serious issues limiting APT from offering true atomic resolution analyses. Instrumentation advances will continue to incrementally improve the situation, but this goal will not be achieved in the near future via technical advances alone. In the present study, we propose a new analytical approach that blends experiment with simulation to create a complete and lattice-based atomistic image of the original system. Although the information provided by APT is incomplete, in actuality, the sheer amount of data generated by this technique is its exceptional strength. Millions of atoms are routinely chemically identified and precisely located in 3D in the course of an experiment. Hence, an almost overwhelming amount of statistical information is available and this is the foundation on which we have built our methods. Our strategic approach is outlined step-by-step in Fig. 1 . A crystalline specimen is analysed via APT ( Fig. 1a ), generating a 3D atomic reconstruction of the original atomic configuration ( Fig. 1b ). In the next step, the average local chemical distribution within the reconstruction is characterized by measuring a set of short-range order (SRO) parameters at increasingly large radii ( Fig. 1c i–iv). SRO parameters are well established for the characterization of chemical correlations in alloyed materials, and we have recently developed an approach to derive these measurements from APT data [22] . It was also demonstrated that SRO measured via APT can provide a quantitative description of the nanostructure present in the system despite its aforementioned limitations. 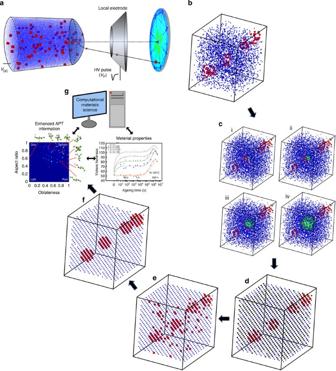Figure 1: Approach for corrected and completed atom probe data. (a) Schematic of atom probe experiment. (b) Close-up of a very small subvolume of APT reconstruction. Small blue spheres represent matrix atoms and large red spheres are solute atoms. (c) SRO is measured by characterization of the local neighbourhood surrounding each atom for increasingly large radii (i–iv). (d) Reconstruction is lattice rectified. The positions of vacant lattice sites due to limited detection efficiency in the experiment are highlighted by black squares. (e) Atoms are replaced at random into the vacant sites while maintaining the original bulk composition. (f) SRO measured incis re-established by swapping positions of restored atoms in a MC simulation. (g) Resulting data informs computational materials science. Figure 1: Approach for corrected and completed atom probe data. ( a ) Schematic of atom probe experiment. ( b ) Close-up of a very small subvolume of APT reconstruction. Small blue spheres represent matrix atoms and large red spheres are solute atoms. ( c ) SRO is measured by characterization of the local neighbourhood surrounding each atom for increasingly large radii (i–iv). ( d ) Reconstruction is lattice rectified. The positions of vacant lattice sites due to limited detection efficiency in the experiment are highlighted by black squares. ( e ) Atoms are replaced at random into the vacant sites while maintaining the original bulk composition. ( f ) SRO measured in c is re-established by swapping positions of restored atoms in a MC simulation. ( g ) Resulting data informs computational materials science. Full size image On further statistical analyses, in many cases, it is observed that significant crystallographic information has been retained in the reconstruction [23] , [24] , [25] ( Supplementary Fig. 2 ). This is discussed in more detail in Supplementary Note 1 . This information can be used to correct the data, atom by atom, to the perfect lattice configuration of the original specimen [26] , [27] ( Fig. 1d ). We term this process lattice rectification. In the rectified data, it will be apparent that there are a substantial number of vacant lattice sites. As a first approximation, it is assumed that this is due solely to a limited detection efficiency, which, in a stochastic manner, effectively omits a significant fraction of the ions field evaporated from the specimen. Atoms can then be replaced into the APT data by filling the vacant sites, and these will be termed restored atoms. The chemical identity of individual restored atoms is chosen at random but with the constraint that after all vacant lattice sites have been filled, the overall composition of the original reconstruction has been maintained ( Fig. 1e ). It is clear from comparing the respective chemical distributions in Fig. 1d,e that most of the restored solute atoms have been placed in incorrect lattice sites. This is also reflected in a drastic change in values when the SRO parameters are re-measured because we are randomly adding atoms to a reconstruction that has significant short-range ordering. At this point, the reconstruction is seeded directly into to a MC algorithm. This MC simulation is specifically adapted such that instead of utilizing interaction potentials, trial moves are accepted or rejected based on their effect on the overall SRO of the system. The SRO parameters measured in the original reconstruction ( Fig. 1c ) are used by the simulation as target values. Atomic positions continue to be swapped at random until the SRO target values have been restored [28] . A critical constraint applied to this simulation is that the positions of the original (experimentally detected) atoms are not moved from their lattice-rectified positions, only the positions of the restored atoms are swapped. The final result is a 3D lattice-based and atomically complete representation of the nanostructure present in the original experimental specimen ( Fig. 1f ). Replacing atoms missing in simulated systems There is no way of confirming the chemical identities of the actual ions lost in the experiment due to detection efficiency; hence, computer-generated APT-like systems provide an excellent means to test the accuracy of our approach for predicting the missing atoms. A range of systems were simulated, each incorporating its own unique nanostructure. In the first case, a series of three ternary ( A–B–C ) systems was simulated on a face-centred cubic lattice. In these simulations, the B -type solute atoms occurred exclusively in spherical precipitates, while the C -type solutes occurred randomly throughout the matrix. An example of these simulations is presented in Fig. 2a . The effect of randomly removing 63% of atoms from the system, to model the effects of detection efficiency in a reflectron-fitted atom probe, is demonstrated in Fig. 2b . The generalized-multicomponent SRO (GM-SRO) parameters were then measured by characterizing the chemical distribution within each of the first five crystallographic shells around every atom [22] . The now-vacant sites on the lattice represent the positions of undetected atoms. Atoms with randomly chosen chemical identities were then restored to these vacant sites as shown in Fig. 2c , while maintaining the overall composition of the system. The data were then seeded directly into the MC simulation, and the originally measured values of the GM-SRO parameters were re-established by swapping the positions of the restored atoms. The final result is presented in Fig. 2d , in which overwhelmingly the solute atoms have been returned correctly to the precipitates. 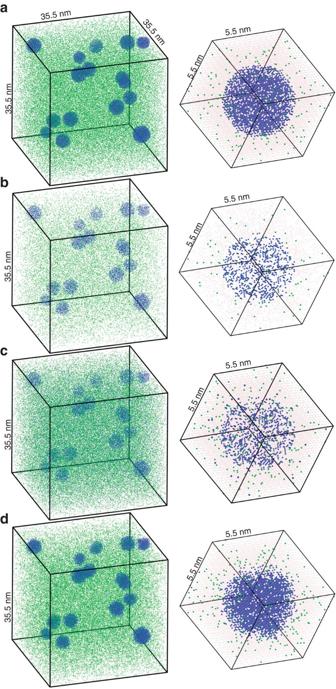Figure 2: Restoring atoms to simulated system. (a) On left is the original simulation (B-type atoms are blue dots, C-type atoms are green and matrix atoms are not shown at this scale for sake of visual clarity). On right is a close-up of a specific precipitate. Matrix atoms are now shown and are now depicted by red dots. (b) Same simulation after 63% of atoms have been removed at random. On right is corresponding close-up of same precipitate. (c) Atoms are replaced at random in the vacant lattice sites. The overall composition of the system has been maintained. (d) The final system after distribution of the restored atoms is rearranged via MC simulation to return the original SRO. Figure 2: Restoring atoms to simulated system. ( a ) On left is the original simulation (B-type atoms are blue dots, C-type atoms are green and matrix atoms are not shown at this scale for sake of visual clarity). On right is a close-up of a specific precipitate. Matrix atoms are now shown and are now depicted by red dots. ( b ) Same simulation after 63% of atoms have been removed at random. On right is corresponding close-up of same precipitate. ( c ) Atoms are replaced at random in the vacant lattice sites. The overall composition of the system has been maintained. ( d ) The final system after distribution of the restored atoms is rearranged via MC simulation to return the original SRO. Full size image Supplementary Note 2 describe how the approach was also successfully applied to systems containing more complicated nanostructures, including precipitates with an ordered structure (for example, L1 2 in Supplementary Fig. 3 ) and features with non-spherical geometries (for example, disc-shaped Guinier–Preston zones in Supplementary Fig. 4 ). The results demonstrate that based on the existing, but incomplete data, not only were atoms accurately replaced back into a precipitate, but also the existing long-range order and shape of these nanostructural features were preserved. It emphasizes the fact that the different crystallographic shells surrounding each atom inherently contain information about the site occupation of elements along different crystallographic orientations. Application to experimental data This approach was then applied to replace the missing atoms in actual experimental APT data. A thermally treated Al-5.6Ag-0.84Cu (at. %) alloy analysis was chosen for this investigation since it contains a significant amount of nanostructure in the form of spherical, coherent Ag Guinier–Preston zones ( Fig. 3a ; Supplementary Fig. 1 ). The data were obtained on a straight-flight path local electrode atom probe 3000X Si. Multiple sets of crystallographic planes in the data were identified and characterized using spatial distribution maps [29] ( Supplementary Fig. 2 ). The precision of both the SRO measurement and the lattice rectification procedure is dependent on the spatial resolution of the APT data to which they are applied. Hence, a 20 × 20 × 100 nm region of interest (ROI), containing 1.2 × 10 6 atoms, free of significant reconstruction artefacts was then identified and isolated. These data are shown in Fig. 3a where at this scale only solute atoms are shown. A close-up within this ROI is also presented in which all the atoms (matrix and solute) are shown. 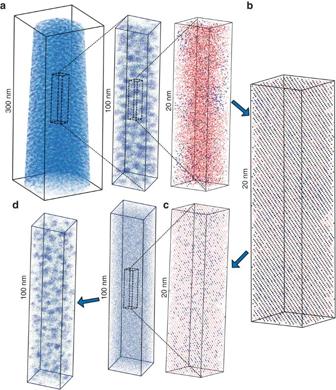Figure 3: Restoring missing atoms to actual APT data. (a) Left, Al-5.6Ag-0.84Cu (at. %) APT reconstruction. ROI is highlighted, which contains 1.2 × 106 atoms. Only solute atoms (Ag blue, Cu green) are shown for clarity. Close-up within ROI also indicates position of matrix ions (Al red). (b) Close-up of ROI after lattice rectification, restoring face-centred cubic crystal. Vacant lattice sites are highlighted by black squares. (c) Close-up of positions of atoms randomly restored atoms to vacant sites. Corresponding image of entire ROI indicates the homogenous distribution of the restored solute atoms. (d) ROI distribution of the restored atoms after the MC simulation to restore SRO. Figure 3: Restoring missing atoms to actual APT data. ( a ) Left, Al-5.6Ag-0.84Cu (at. %) APT reconstruction. ROI is highlighted, which contains 1.2 × 106 atoms. Only solute atoms (Ag blue, Cu green) are shown for clarity. Close-up within ROI also indicates position of matrix ions (Al red). ( b ) Close-up of ROI after lattice rectification, restoring face-centred cubic crystal. Vacant lattice sites are highlighted by black squares. ( c ) Close-up of positions of atoms randomly restored atoms to vacant sites. Corresponding image of entire ROI indicates the homogenous distribution of the restored solute atoms. ( d ) ROI distribution of the restored atoms after the MC simulation to restore SRO. Full size image Next, the complete set of GM-SRO parameters, [α Al–Al , α Al–Ag , α Al–Cu , α Ag–Al ,…, α AlAgCu–AlCu , α AlAgCu–AgCu ], was measured for the first five crystallographic shells where α AB–CD represents the distribution of C- and D- type atoms around A - and B- type atoms. A key assumption that we make is that ion detection is effectively a stochastic process, and hence, although a significant fraction of atoms are missing from the final reconstruction, this does not affect the values of the measured SRO, that is, the SRO we measure from a data set with 57% detection efficiency is the same as that which would be measured in a hypothetical 100% detection efficiency data set. The validity of this assumption has been previously investigated [28] . It is also well known that in certain analyses can occur a non-stochastic loss of ions due to a combination of preferential evaporation and detector pile-up effects [30] , [31] , however, this is not expected to be a significant issue for the alloys chosen for this study. Following this, the ROI was subject to lattice rectification. It has previously been estimated that in a reasonable-sized subvolume of a pure Al reconstruction upwards of 85% of the rectified atoms is returned to their correct lattice sites [26] . The effect of restoring the lattice is clearly apparent when comparing the close-ups in Fig. 3a,b . The vacant lattice sites were then identified and their positions are highlighted in Fig. 3b by black squares. As for the simulations described above, atoms were restored to these vacant sites, their chemical identities chosen at random but with the constraint that the overall bulk composition remained the same throughout this process. A close-up of the restored atoms is shown in Fig. 3c . The corresponding image of the entire subvolume indicates the homogeneous distribution of the restored solute atoms throughout the system, and is in clear contrast to the distribution of the experimentally detected solutes in Fig. 3a . The entire data set (including both detected and restored atoms) was seeded into the MC simulation with target SRO based on the measured GM-SRO parameters that measured the original APT data. The final solute distribution of the restored atoms is presented in Fig. 3d . There is a striking agreement between the distribution of the detected and restored solute atoms. This is as expected, since they effectively represent two halves of the same material system that has been randomly split through the action of the microchannel plate detector system. Supplementary Fig. 5 shows a further example where this technique has been equally effective in restoring APT data containing precipitates with more complicated shapes. The final data set is a hybrid of experimental and simulated data, an approximation of a completed 3D image of the original specimen in which every atom is accounted for chemically and spatially. APT-informed DFT calculation There are many ways that the atomically complete hybrid APT data can potentially be used to inform simulations. The simplest example is a direct comparison between the nature and distribution of nanostructure characterized in the completed experimental data and that predicted by simulation. Alternatively, the hybrid APT data set could potentially actually be directly seeded into a kinetic MC or MD simulation to predict how the system will evolve with time, when subject to specific treatments or conditions. Here we implement DFT simulations to demonstrate local area energy mapping in the thermally treated Al-5.6Ag-0.84Cu (at. %) system presented in Fig. 3 . DFT simulation was chosen because it can in principle predict energetic, electronic and elastic properties of a specific atomic configuration. It is easy to envisage that local compositional variation will impact local properties, and then the macro-properties. However, precise quantification of realistic structures to undertake such a calculation is a grand challenge—hindering a true material optimization at the atomic level. To demonstrate this concept, we have carried out DFT simulations to calculate ‘local cohesive energy’, ‘local Fermi energy’ and ‘local elastic moduli’ within regions of the specimen. The cohesive energy is closely correlated with many properties, including interatomic bonding strength, molar volume and compressibility [32] , while the Fermi energy is critically important for the electrical and thermal properties of solids [33] . To conduct the energy mapping, first, 49 groups of ‘cubic’ 32-atom (2 × 2 × 2 supercells) subvolumes were randomly sampled from the hybrid APT data, as illustrated in Fig. 4a . Then, the duplicity of these subvolumes was assessed, indicating 15 pure Al subvolumes and 8 subvolumes containing only a single Ag atom. In total, 25 unique configurations were identified, and these are presented in Fig. 4 . To account for environmental effects and enable periodic boundary conditions, each unique 32-atom configuration was then embedded into a 108-atom 3 × 3 × 3 supercell. DFT total energy calculations were subsequently performed, allowing atomic relaxation, that is, possible structural distortions were taken into account. 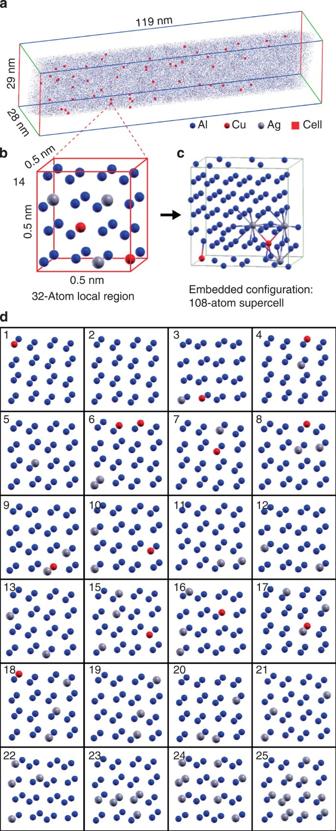Figure 4: Sampling regions of the hybrid APT data for local property mapping. (a) Slice of the hybrid APT data, red squares indicate regions that have been randomly sampled. (b) Close-up of one of the sampled 32-atom subvolumes. (c) The subvolume inbembedded into a 108-atom supercell. (d) The unique 32-atom configurations. The sequence in which these configurations appear in this figure is based on the associated increase in cohesive energy calculated inFig. 5. Figure 4: Sampling regions of the hybrid APT data for local property mapping. ( a ) Slice of the hybrid APT data, red squares indicate regions that have been randomly sampled. ( b ) Close-up of one of the sampled 32-atom subvolumes. ( c ) The subvolume in b embedded into a 108-atom supercell. ( d ) The unique 32-atom configurations. The sequence in which these configurations appear in this figure is based on the associated increase in cohesive energy calculated in Fig. 5 . Full size image The calculated local cohesive energy as a function of number of Ag atoms contained in each subvolume is presented in Fig. 5a . Local cohesive energy clearly decreases with a linear dependence on increasing number of local Ag atoms (goodness of fit of linear regression r 2 =0.98). The ~0.1 eV per atom variation of cohesive energy across the Ag concentration range considered here is relatively small (that is, within the error range for standard DFT calculation for a given system). However, our systematic study consistently consolidates the reliability of this trend. Indeed, by examining two higher-concentration configurations, 32-Ag-atom and 108-Ag-atom, it has been confirmed that this linearity is still valid. Such behaviour is reasonable if one compares the cohesive energy values of bulk Al and Ag. Experimental values are 3.39 eV per atom for pure Al versus 2.95 eV per atom for pure Ag [34] and the corresponding values calculated in this study are 3.33 eV per atom and 2.56 eV per atom, respectively. In the calculations performed here, for a single Al and Ag atom, the spin polarisation and Hund’s effects were explicitly included. It is also notable that, for each Ag concentration, increasing the number of Cu atoms tends to increase the local cohesive energy, indicating an attractive interaction between Ag–Cu atoms. 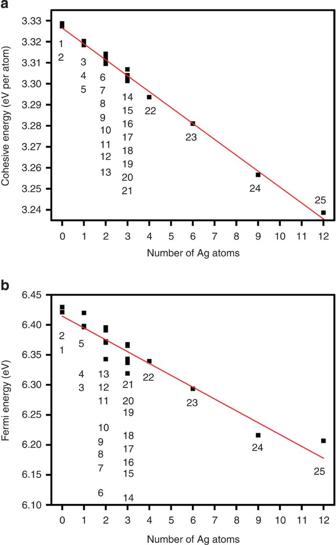Figure 5: DFT calculation of local energies as a function of Ag content. (a) Local cohesive energy and (b) local Fermi energy calculated for each unique 32-atom configuration. Figure 5: DFT calculation of local energies as a function of Ag content. ( a ) Local cohesive energy and ( b ) local Fermi energy calculated for each unique 32-atom configuration. Full size image The calculated local Fermi energy as a function of number of Ag atom is presented in Fig. 5b . Again, with increasing the Ag concentration, the Fermi energy decreases. The graph demonstrates that the local addition of Cu atoms further decreases the local Fermi energy (goodness of fit of linear regression r 2 =0.90). This behaviour is to be expected since the Fermi energies of Ag and Cu are much smaller than that of Al. Experimental values are 5.49 eV for Ag, 7.00 eV for Cu and 11.7 eV for Al (ref. 33 ). The results demonstrate the importance of characterizing and controlling the local microstructure to tailor the micro- and ultimately macro-properties accordingly. The final DFT example presented in this study uses the information in the unique hybrid APT data format to investigate the local mechanical and thermodynamic properties. In this case, the central parameters, namely, the elastic constants, are derived by applying a set of homogeneous deformations and calculating from the second derivative of the total energy as a function of volume, tetragonal and trigonal lattice distortions around the equilibrium structures. To our knowledge, a systematic comparison of elastic quantities as a function of local microstructure variation has not been previously reported. Due to the low symmetries involved, we have selected seven of the 32-atom configurations in Fig. 4 , whose relaxed equilibrium cells are tetragonal (or cubic) structures. For these cases, expressions can be derived for bulk modulus, shear modulus and Young’s modulus, Values for the six independent elastic constants have been calculated and are listed in Table 1 . The resulting measurements of local elastic quantities are presented in Fig. 6 , again plotted as a function of the number of Ag atoms. Table 1 Local elastic constants calculated within 32-atom subvolume configurations. 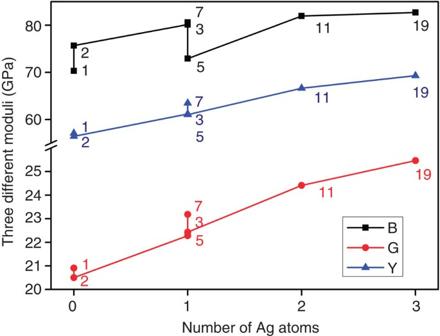Figure 6: Local bulk modulus (B), shear modulus (G) and Young's modulus (Y). Moduli calculated by DFT simulations informed directly by local regions of the hybrid APT reconstruction and plotted as a function of Ag content. Full size table Figure 6: Local bulk modulus (B), shear modulus (G) and Young's modulus (Y). Moduli calculated by DFT simulations informed directly by local regions of the hybrid APT reconstruction and plotted as a function of Ag content. Full size image First, from Table 1 it is apparent that all calculated elastic constants satisfy the criteria of mechanical stability for tetragonal crystals [35] : C 11 >0, C 33 >0, C 44 >0, C 66 >0, ( C 11 − C 12 )>0, ( C 11 + C 33 −2 C 13 )>0 and [2( C 11 + C 12 )+ C 33 +4 C 13 ]>0. Hence, it can be asserted that all the examined local configurations are intrinsically stable. Further, the general trend for each of these three moduli ( B , G and Y ) is similar, increasing with Ag concentration. Yet, for a given Ag concentration, the calculated order of moduli values varies. All the three moduli ( B , G and Y ) can be used to evaluate material hardness, however, G and Y are better indicators [36] . The calculated B , G and Y values (75.67, 20.51 and 56.42 GPa, respectively) for pure Al agree reasonably well with those derived experimentally (76, 26 and 70 GPa). The calculations presented in Fig. 6 results consistently suggest that adding Ag will increase the local hardness. Microscopy has continued to make great strides in characterizing material microstructure with ever increasing details. However, there still remains an intrinsic disconnect between the microstructure and the bulk material properties. The way in which local microstructure variations influence the macro-property is poorly understood, restricting the potential to use information generated by microscopy for the purpose of materials’ design. Hence, the aim of this study is twofold: first, from a microscopy perspective, the goal has been to extend the current limits of APT by generating complete hybrid experimental-analytical data sets of a form that can be seeded directly into atomistic simulations. Second, from the perspective of physical material properties, by using these hybrid data sets, we attempt to bridge the gap between microstructure and macro-properties by studying the local properties. The significance of this is that collectively these local properties will contribute to define to the macroscopic properties. For inhomogeneous systems, in many cases, the ability to accurately probe the local properties is highly desirable and represents a crucial step to understand the normally complicated bulk properties and to offer information for material design [37] , [38] . The results demonstrate the importance of characterizing and controlling the local microstructure to tailor micro- and ultimately macro-properties accordingly. It must be noted that the method that has been developed to restore the data missing from APT characterization is based on a statistical process. The exact configuration of solute atoms that converges to a particular set of SRO parameters is not necessarily unique. Hence, the hybrid APT data set that is ultimately generated is one of the number of possible atomic configurations that could be obtained. However, this is analogous to examining two or more successive APT analyses of the same specimen (for example, a solid solution). Although the individual distributions of solutes will be statistically equivalent, at the atomic scale, identical configurations would never be observed. Hence, the hybrid APT data represents the most likely configuration of atoms based on the existing experimental information, which, although not unique, is a highly accurate representation of the true atomic structure of the material. The approach also makes several key assumptions and approximations. These are acknowledged here to map out the challenges for routine and meaningful rectification and restoration of APT data into the future: it is assumed that detection efficiency is independent of ionic identity; data must be free of aberrant regions of high and low density; and the SRO analysis must have sufficient statistics to ensure that measurements are not unduly biased and are representative of the bulk system. Currently, all atoms are mapped back onto a perfect single crystal lattice by the rectification process. Hence, the alloy systems studied in this work were either solid solutions of engineering significance or alloy systems where precipitates are coherent with the surrounding matrix. The understanding gained from relatively simple systems is instrumental in defining the pathways to develop the infrastructure to investigate complex systems containing, for instance, interstitial atoms, defects, secondary phases or even grain boundaries. We envisage that this will be a future development of the methodology, which will require development of secondary corrections based on all of the available information. Most of the limitations listed above are issues affecting all APT-based characterizations, not just those developed in this study. As such, research is already ongoing towards limiting the influence of all of these effects. Indeed, instrumentation will undoubtedly continue to improve and rather than being relegated by such advances, the analytical approach described here will be complemented by these developments progressively improving accuracy and applicability. The APT-based methods developed in this study represent a bridge between microstructure and micro-property. This outlook opens the pathway for a formidable nexus between the determination of the structure of a material and its properties by using a range of other atomistic simulations (such as MC and MD), particularly for intrinsically highly inhomogeneous systems. One could also conceive of large-scale orbital-free DFT [39] so as to relax the hybrid atom probe data and circumvent the limitation currently associated with the hard lattice originating from the rectification procedure, which could be of paramount interest for replacing interstitial atoms or obtain the appropriate local crystal structure of precipitates, for example, allowing for comparison with other characterization techniques such as electron microscopy or X-ray or neutron scattering. Atom probe experiments Al-5.6Ag-0.84Cu (at. %) alloy samples were solution treated for 1 h at 525 °C in a salt bath and cold water (15–20 °C) quenched. Specimens for APT were prepared first by cutting small blanks (0.3 mm × 0.3 mm × 15 mm) from the bulk alloy material before thermal ageing. Needle-shaped specimens for APT analysis, with radii ~50 nm, were prepared using standard two-stage electropolishing techniques [4] . APT analysis was performed using a local electrode atom probe 3000X Si manufactured by Cameca. Experiments were performed at a specimen temperature of ~20–25 K under ultrahigh vacuum conditions of ~1 × 10 −8 Pa, in voltage-pulsing mode with a pulse fraction of 20% and a pulse repetition rate of 200 kHz. Reconstruction of the APT data was performed using the IVAS software package, which is based on a reverse-projection algorithm [40] , and was calibrated using techniques developed by Gault et al. [41] , [42] SRO-based MC simulations The first step in our process after acquiring and reconstructing the atom probe data is to characterize the average local chemical distribution via the measurement of SRO parameters. The GM-SRO [22] is based on the probability of finding particular types of atoms around another atom defined as Taking the example of an Al–Ag–Cu alloy, represents the probability of finding a Cu atom in the first shell ( m=1 ) around an Ag atom. Likewise, represents the probability of finding an Ag or Cu atom in the third crystallographic shell around Cu atom. The resulting GM-SRO expression is given by where equals 1 if the two sets contain exactly the same atomic species and 0 otherwise, and . Again taking the current example, this results in a set of possible parameters where each element of this set can be measured as a function of radius, m . This represents a comprehensive statistical description of the system. An approach for measuring GM-SRO in APT reconstructions, taking into account its finite spatial resolution and limited detected efficiency, has previously been developed [22] . It has previously been demonstrated that in many cases, the SRO contains sufficient information to accurately predict the identities of the atoms missing due to finite detection in an APT experiment [28] . MC approaches have previously been developed to drive a simulated atomic system to a specific configuration based on using experimentally measured SRO as target parameter [28] , [43] . Starting at some initial configuration atoms in a lattice, in each step of an SRO-based MC simulation, the relative positions of two atoms are swapped at random. After each trial move, the set of SRO is re-evaluated and if the swap drives these parameters towards their target values the move is accepted, otherwise it is rejected and the atoms are replaced to their original positions. Defining whether or not the swapping of a pair of atoms has improved the overall configuration of the system is not straightforward. The target SRO can potentially comprise a large set of parameters. Taking the example above, it is possible that the action of randomly swapping a pair of atoms may move the system towards the target but simultaneously also move the system away from the target. Hence, an objective metric is required in the algorithm to decide on whether the trial move has either improved or worsened the overall atomic configuration. Here, we define residual as a measure of the difference in the instantaneous SRO in the simulated system and the experimentally measured target SRO values (denoted by the prefix T ): A swap reducing the value of Δ SRO is automatically accepted. The required number of trial moves is dependent on the magnitude of the difference between the target and the current actual SRO parameter values, the concentration of each element, number of crystallographic shells, size of the data set and the number of elements that constitute the alloy. Lattice rectification In APT, crystallographic information is most apparent in the form of crystallographic planes. Spatial distribution maps provide an efficient approach for the characterization of these atomic planes ( Supplementary Fig. 2 ), in terms of inter-planar spacing, orientation and resolution (that is, the accuracy to which atoms are placed on these planes). Knowledge of this underlying lattice structure combined with the local distribution of atoms in the raw data facilitates the remapping of the perturbed atom positions back to their true lattice sites, a process that we termed lattice rectification [26] . Having identified the orientation of a set of crystallographic planes { hkl }, it can be inferred that in the specimen, any two neighbouring atoms were actually separated by a distance corresponding to an exact multiple of the plane spacing in this direction. A small correction can be applied to the reconstructed coordinates of atoms to satisfy this condition. If three independent sets of planes are identified within the data, this correction of atoms onto the closest plane, simultaneously in three directions, provides a unique solution, that is, a single lattice site. The significance of this result is that the lattice structure of the specimen is recovered via a progressive atom-by-atom triangulation. The smallest possible correction is being made to the atomic coordinates, requiring access to highly spatially resolved data. However, trajectory aberrations can result in significant inaccuracies in the original 3D positioning of an atom. Trajectory aberrations most often originate primarily from local magnification effects on the specimen surface arising from either the preferential evaporation or retention of certain atoms. Such aberrations cause two main issues: (1) the crystalline lattice appears smeared out by small dithering of the atomic positions and (2) the shape of larger features (that is, precipitate, layers and so on) appears distorted. These effects have been thoroughly described in the literature, including in recent reviews on the topic [44] , [45] , [46] . However, as shown in this study, it is often possible to identify high-quality subvolumes of the data devoid of significant local magnification effects. This simple lattice rectification approach requires APT reconstructions within which sufficient crystallographic information can be identified, and incorporate significant regions of interest free of aberrations. It is noted that this is currently not the case for many complex systems now studied by APT. Although some of these contain a significant amount of crystallographic information [47] , until the accuracy the original reconstruction can be improved, lattice rectification is not meaningful for these systems. DFT simulations All-electron DFT calculations were performed using the generalized gradient approximation [48] with the DMol3 program package [49] . The wave functions were expanded in terms of a double-numerical quality basis set, with a set of large values of real-space cut-off (Cu: 9.45 Bohr; Ag: 9.98 Bohr; Al: 10.88 Bohr). A reciprocal space of 4 × 4 × 4 K -point meshes was employed in the calculations of the 108-atom supercells. How to cite this article: Moody, M. P. et al. Atomically resolved tomography to directly inform simulations for structure-property relationships. Nat. Commun. 5:5501 doi: 10.1038/ncomms6501 (2014).